Direct conversion of mouse and human fibroblasts to functional melanocytes by defined factors Direct reprogramming provides a fundamentally new approach for the generation of patient-specific cells. Here, by screening a pool of candidate transcription factors, we identify that a combination of the three factors, MITF, SOX10 and PAX3, directly converts mouse and human fibroblasts to functional melanocytes. Induced melanocytes (iMels) activate melanocyte-specific networks, express components of pigment production and delivery system and produce melanosomes. Human iMels properly integrate into the dermal–epidermal junction and produce and deliver melanin pigment to surrounding keratinocytes in a 3D organotypic skin reconstruct. Human iMels generate pigmented epidermis and hair follicles in skin reconstitution assays in vivo . The generation of iMels has important implications for studies of melanocyte lineage commitment, pigmentation disorders and cell replacement therapies. Melanocytes are neural crest-derived pigment-producing cells localized at the basal layer of epidermis and hair follicles. Melanocytes synthesize melanin pigment within specialized lysosome-related structures known as melanosomes. Melanin pigment is then transferred to adjacent keratinocytes to form pigmented skin or hairs, protecting skin from ultraviolet irradiation [1] . Loss of melanocytes in the skin (vitiligo) affects 0.1% to greater than 8% population worldwide and depigmentation may be the source of severe psychological distress, diminished quality of life and increased risk of psychiatric morbidity [2] . Autologous melanocyte transplantation is effective in treating stable vitiligo. However, it is not widely clinically used due to issues such as donor site infection, scar or irregular pigmentation [3] . Therefore, there is an unmet clinical need to efficiently generate scalable amount of autologous melanocytes. The discovery that fibroblasts can be directly reprogrammed into muscle cells and neurons by combinations of lineage-enriched transcription factors [4] , [5] , [6] , [7] , [8] , [9] , [10] , [11] leads us to hypothesize that melanocytes can be generated directly from fibroblasts without going through a pluripotent state. Previous studies have demonstrated a critical role of microphthalmia-associated transcription factor (MITF) in melanocyte linage determination from neural crest cells [12] and forced expression of MITF in NIH3T3 fibroblasts converted them into melanocyte-like cells [13] . However, such induced cells expressed only some of the melanocyte-specific markers and lacked functional characteristics of melanocytes [13] . Here, by screening a pool of candidate transcription factors, we discover that the three factors, SOX10, MITF and PAX3, are sufficient to directly reprogram human and mouse fibroblasts to melanocytes. Induced melanocytes (iMels) acquire phenotypical and functional characteristics of normal melanocytes. Generation of functional melanocytes by direct reprogramming methods provides a potential source for autologous melanocytes to treat skin pigmentation disorders. 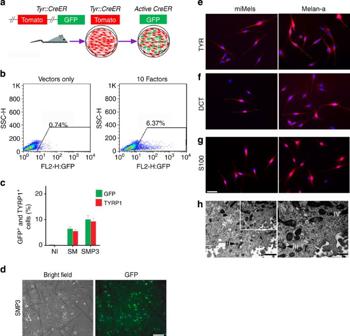Figure 1: Screening for melanocyte direct reprogramming factors. (a) Scheme for melanocyte direct reprogramming transcription factor (TF) screening. Screening was performed using fibroblasts from theTyrosinase-CreER/Gt(ROSA)26Sortm4(ACTB-tdTomato,-EGFP)Luo/J mice. When tyrosinase (TYR) was activated, Cre activation resulted in excision of the tomato cassette and expression of GFP in the presence of 4-HT. (b) Flow cytometric analysis of the GFP+cells after cells were infected with viruses packaged with 10 candidate factors (right panel) or vector only (left panel). (c) Flow cytometric analysis of GFP and TYRP1 expressions after cells were infected with control vectors (NI), SOX10 and MITF (SM) or SOX10, MITF and PAX3 (SMP3). Representative data are from three independent experiments. (d) Morphology of FACS-sorted GFP+cells. Mouse fibroblasts were infected with SMP3 and sorted based on GFP expression at day 14. Scale bar, 50 μm. (e–g) Immunostaining analysis of mouse induced mouse melanocytes (miMels) using antibodies specific for TYR (e), DCT (f) and S100 (g). Secondary antibody was labelled with Alexa Fluro 594. DAPI was used to stain the nuclei. Melan-a mouse melanocytes were used as a positive control. Scale bar, 30 μm. (h) Electron microscopy analyses showed that miMels contained many mature melanosomes in the cytoplasm. Arrow heads point to the different stages of melanosomes, including stage II, III and IV. Scale bar, 400 nm (left panel) and 200 nm (right panel). Screening for melanocyte-reprogramming factors Reasoning that multiple transcription factors would probably be required to reprogram fibroblasts into functional melanocytes, we selected 10 candidate transcription factors that are related to neural crest lineage determination and melanocyte differentiation ( Supplementary Table 1 ) [12] , [14] , [15] , [16] , [17] , [18] , [19] , [20] . To efficiently monitor melanocyte differentiation by flow cytometric analysis, we developed a transcription factor screening assay using tail fibroblasts (TTFs) from Tyrosinase-CreER ; Gt(ROSA)26Sor tm4(ACTB-tdTomato,-EGFP)Luo /J reporter mice [21] . Tyrosinase (TYR)-driven CreER expression in melanocytes converts these mouse cells from expressing red fluorescent protein to green fluorescent protein (GFP) on treatment with 4-hydroxytamoxifen (4-HT). This makes it possible to monitor the emergence of TYR-positive (TYR + ) melanocytes by detecting GFP expression ( Fig. 1a ). Retroviruses carrying 10 candidate mouse transcription factors were prepared and a mixture of all the factors was used to infect the TTFs. Expression of transgenes was confirmed by quantitative reverse transcription PCR (qRT–PCR; Supplementary Fig. 1 ) and virus packaged with vector only was used as a negative control. Twelve days after infection with all factors, GFP-positive (GFP + ) cells were observed in the presence of 4-HT ( Fig. 1b ), indicating activation of the TYR promoter in cells. Significantly fewer GFP + cells were detected in the control, vector-only cells ( Fig. 1b ). Next we sought to determine the minimal set of genes required for melanocyte induction from fibroblasts. Given the known dominant role of SOX10 during neural crest lineage differentiation, SOX10 was introduced into TTFs combined with every other single factor first. The greatest number of GFP + cells was produced when SOX10 was combined with MITF ( Supplementary Fig. 2a ). However, the SOX10/MITF combination elicited modest reprogramming efficiencies with GFP + cells comprising 6.44% of all cells. Therefore, we added a third transcription factor (from the eight remaining) and analysed the percentage of GFP + cells using each combination. SOX10/MITF/PAX3 and SOX10/MITF/SOX9 combinations increased the generation of GFP + cells, compared with other combinations ( Supplementary Fig. 2b ). The addition of a fourth factor to the SOX10/MITF/PAX3 or SOX10/MITF/SOX9 combinations failed to further increase the percentage of GFP + cells ( Supplementary Fig. 4b ), including SOX10/MITF/PAX3/SOX9 combination ( Supplementary Fig. 2c ). To further confirm melanocytic reprogramming, we examined the percentage of TYRP1-positive (TYRP1 + ) cells using flow cytometric analysis after reprogramming with different combinations of transcription factors. The results demonstrated that the SOX10/MITF/PAX3 combination induced the highest percentage of TYRP1 + cells ( Supplementary Fig. 3 ). Statistical analysis showed that the SOX10/MITF/PAX3 combination activated higher GFP and TYRP1 expressions, compared with other combinations ( Fig. 1c ; Supplementary Fig. 4a ). Therefore, melanocytes induced by SOX10/MITF/PAX3 (SMP3) were characterized in additional studies. Figure 1: Screening for melanocyte direct reprogramming factors. ( a ) Scheme for melanocyte direct reprogramming transcription factor (TF) screening. Screening was performed using fibroblasts from the Tyrosinase-CreER / Gt(ROSA)26Sor tm4(ACTB-tdTomato,-EGFP)Luo /J mice. When tyrosinase (TYR) was activated, Cre activation resulted in excision of the tomato cassette and expression of GFP in the presence of 4-HT. ( b ) Flow cytometric analysis of the GFP + cells after cells were infected with viruses packaged with 10 candidate factors (right panel) or vector only (left panel). ( c ) Flow cytometric analysis of GFP and TYRP1 expressions after cells were infected with control vectors (NI), SOX10 and MITF (SM) or SOX10, MITF and PAX3 (SMP3). Representative data are from three independent experiments. ( d ) Morphology of FACS-sorted GFP + cells. Mouse fibroblasts were infected with SMP3 and sorted based on GFP expression at day 14. Scale bar, 50 μm. ( e – g ) Immunostaining analysis of mouse induced mouse melanocytes (miMels) using antibodies specific for TYR ( e ), DCT ( f ) and S100 ( g ). Secondary antibody was labelled with Alexa Fluro 594. DAPI was used to stain the nuclei. Melan-a mouse melanocytes were used as a positive control. Scale bar, 30 μm. ( h ) Electron microscopy analyses showed that miMels contained many mature melanosomes in the cytoplasm. Arrow heads point to the different stages of melanosomes, including stage II, III and IV. Scale bar, 400 nm (left panel) and 200 nm (right panel). Full size image Characterization of mouse iMels We monitored the GFP + cell population daily under a fluorescence microscope after TTFs derived from Tyrosinase(TYR)-CreER / Gt(ROSA)26Sor tm4(ACTB-tdTomato,-EGFP)Luo /J mice were infected with virus carrying the SMP3 combination. GFP + cells with melanocytic morphology emerged 14 days after induction ( Fig. 1d ; Supplementary Fig. 5a,b ). Most of the sorted GFP + cells showed TYR expression by fluorescence-activated cell sorting (FACS; Supplementary Fig. 5c ) and expressed the protein components of pigment production and delivery machineries including TYR, DCT, Melan-A and SILV ( Fig. 1e,f ; Supplementary Fig. 6a ) by immunocytochemistry. We also observed that S100, a calcium-binding protein, is highly expressed in the induced cells ( Fig. 1g ). Transcriptional analysis by RT–PCR revealed the expression of multiple melanocyte-specific genes, including TYR , TYRP1 , DCT , SILV and P as well as endogenous MITF , SOX10 and PAX3 ( Supplementary Fig. 6b ). Meanwhile, transgenic SOX10 , MITF and PAX3 were still expressed in the GFP + cells ( Supplementary Fig. 6c ). Electron microscopy showed that GFP + -induced cells produced melanosomes at different developmental stages ( Fig. 1h ), including mature melanin-containing (types III and IV) melanosomes. We then tested the SMP3 combination in mouse embryonic fibroblasts (MEFs) and TTFs derived from adult C57BL/6 mice. We found that melanocyte-specific markers including TYR , TYRP1 and DCT were expressed as early as 5 days after MEFs were infected with the SMP3 combination ( Fig. 2a ). Since melanocytes are more resistant to G418 than fibroblasts [22] , we cultured the SMP3-infeced MEFs on layers of XB2 keratinocyte feeder cells for 14 days with G418. G418-resistent cells with typical melanocyte morphology showed strong Dopa activity ( Fig. 2b,c ). The majority of the G418-resistant cells expressed TYR, Melan-A and S100 ( Fig. 2d–f ) and displayed melanocyte-specific gene expression patterns ( Fig. 2g ). Similar results were obtained when adult TTFs were infected with the SOX10, MITF-GFP and PAX3 (SM GFP P3) combination and these adult TTFs expressed melanocytic markers after infection with SM GFP P3 ( Supplementary Fig. 7a ). GFP + cells ( Supplementary Fig. 7b ) were sorted out using FACS and cultured in melanocyte-inducing medium. As expected, the reprogrammed GFP + cells showing typical melanocyte morphologies ( Supplementary Fig. 7c ) displayed higher expression levels of melanocytic markers, compared with adult TTFs infected with vector only ( Supplementary Fig. 7d ). 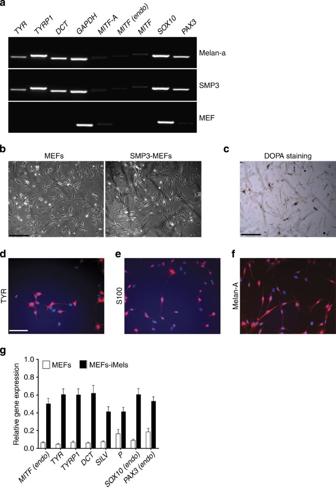Figure 2: Direct reprogramming of MEFs into iMels. (a) RT–PCR analysis of melanocytic markers in MEFs that were reprogrammed by SMP3 combination. MEFs infected with SMP3 were collected for RT–PCR analysis at day 5 after infection. MEFs and melan-a mouse melanocytes were used as negative and positive controls, respectively. The melanocytic markers includedTYR,TYRP1,DCT,MITF(endo),SOX10andPAX3.GAPDHhere was used as an internal control. (b) Morphologies of parental MEFs and SMP3-induced MEFs (SMP3-MEFs). MEFs (left panel) were infected with viruses containing SMP3, cultured for 19 days and then selected under G418 and photographed (right panel). Scale bar, 50 μm. (c) Dopa activity in mouse iMels. Reprogrammed cells were stained by dopamine and showed Dopa activity. Scale bar, 50 μm. (d–f) Immunocytochemical staining of iMels derived from MEFs (MEF-iMels) using antibodies specific for TYR, S100 and Melan-A. Scale bar, 25 μm. (g) qRT–PCR analysis of melanocytic markers, includingMITF(endo),TYR,TYRP1,DCT,P,SOX10(endo) andPAX3(endo) in MEF-iMels and MEFs. Data shown are mean±s.d. of the expression from three independent experiments. Figure 2: Direct reprogramming of MEFs into iMels. ( a ) RT–PCR analysis of melanocytic markers in MEFs that were reprogrammed by SMP3 combination. MEFs infected with SMP3 were collected for RT–PCR analysis at day 5 after infection. MEFs and melan-a mouse melanocytes were used as negative and positive controls, respectively. The melanocytic markers included TYR , TYRP1 , DCT , MITF (endo), SOX10 and PAX3 . GAPDH here was used as an internal control. ( b ) Morphologies of parental MEFs and SMP3-induced MEFs (SMP3-MEFs). MEFs (left panel) were infected with viruses containing SMP3, cultured for 19 days and then selected under G418 and photographed (right panel). Scale bar, 50 μm. ( c ) Dopa activity in mouse iMels. Reprogrammed cells were stained by dopamine and showed Dopa activity. Scale bar, 50 μm. ( d – f ) Immunocytochemical staining of iMels derived from MEFs (MEF-iMels) using antibodies specific for TYR, S100 and Melan-A. Scale bar, 25 μm. ( g ) qRT–PCR analysis of melanocytic markers, including MITF (endo), TYR , TYRP1 , DCT , P , SOX10 (endo) and PAX3 (endo) in MEF-iMels and MEFs. Data shown are mean±s.d. of the expression from three independent experiments. Full size image Direct reprogramming of human fetal dermal fibroblasts into iMels To test whether human fibroblasts can directly be reprogrammed into melanocytes, we infected passaged primary human fetal dermal fibroblasts (fetal hFs) with the human SM GFP P3 combination. SM GFP P3-infected cells were cultured under G418 selection until the cell population with typical melanocyte morphology overwhelmed other cell populations. During this process, we analysed the percentage of TYR + and TYRP1 + cells in the culture using flow cytometric analysis. About 40% of cells with typical melanocyte morphology were observed by day 40 ( Fig. 3a–c ), and the majority of the cells showed typical melanocyte immuno-phenotypes by day 80 ( Fig. 3a,b ). We continued to culture these melanocytic cells and found that 99.3% of the enriched cells were TYR + cells at day 100 ( Fig. 3d ). Except TYR ( Fig. 4a ), hiMels expressed TYRP1, DCT, SILV, S100 and Melan-A ( Fig. 4b–f ). qRT–PCR analysis further confirmed that the melanocyte-specific gene network was activated ( Fig. 4g ). Endogenous expression of PAX3 , SOX10 and MITF was also induced ( Fig. 4g ). Meanwhile, hiMels were capable of producing melanin pigment, as revealed by Fontana–Mason staining ( Fig. 4h ). To further confirm the melanocyte identity, we found that hiMels contained authentic melanosomes from early stage (type II) to mature melanin-containing (types III and IV) melanosomes ( Fig. 4i ). As expected, we found that transgenic PAX3 , SOX10 and MITF were still expressed in hiMels ( Fig. 4j ). Concerned that the melanocyte phenotype and function might be dependent on continued transgene expression, we introduced the viruses that express doxycycline-inducible PAX3, SOX10 and MITF into fetal hFs. Transgenic expression of PAX3 , SOX10 and MITF was induced for 2 weeks and then silenced by withdrawing doxycycline from the culture medium ( Fig. 5a ). The silenced cells were cultured for another 80 days and analysed by qRT–PCR and immunostaining assays. The melanocytic markers continued to be expressed without exogenous PAX3 , SOX10 and MITF expression ( Fig. 5b,c–f ). These data indicate that the induced melanocytic phenotype is stable and independent of transgene expression. 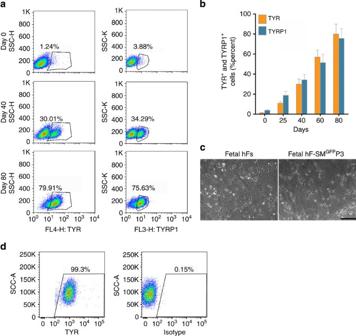Figure 3: Direct reprogramming of human fibroblasts into iMels. (a) Representative flow cytometry plots for analyses of TYR+and TYRP1+cells in SMGFPP3-induced cells at indicated time points. Fetal hFs were infected with SMGFPP3, sorted and selected in the medium containing G418. Cells were collected and flow cytometrically analysed at day 0, 40 and 80. (b) Percentage of TYR+and TYRP1+cells in SMGFPP3-induced cells at indicated time points. Fetal hFs were infected with SMGFPP3, sorted and selected in media containing G418. Cells were analysed by flow cytometry at day 0, 25, 40 and 80. Representative data are from three independent experiments. (c) Cell morphology of fetal hFs and iMels derived from fetal hFs. Representative images of fetal hFs and iMels derived from fetal hFs (fetal hF-SMGFPP3) were photographed at day 40. Scale bar, 50 μm. (d) Representative flow cytometry plots for analyses of TYR+cells after cells were reprogrammed by SMGFPP3 by day 100. Figure 3: Direct reprogramming of human fibroblasts into iMels. ( a ) Representative flow cytometry plots for analyses of TYR + and TYRP1 + cells in SM GFP P3-induced cells at indicated time points. Fetal hFs were infected with SM GFP P3, sorted and selected in the medium containing G418. Cells were collected and flow cytometrically analysed at day 0, 40 and 80. ( b ) Percentage of TYR + and TYRP1 + cells in SM GFP P3-induced cells at indicated time points. Fetal hFs were infected with SM GFP P3, sorted and selected in media containing G418. Cells were analysed by flow cytometry at day 0, 25, 40 and 80. Representative data are from three independent experiments. ( c ) Cell morphology of fetal hFs and iMels derived from fetal hFs. Representative images of fetal hFs and iMels derived from fetal hFs (fetal hF-SM GFP P3) were photographed at day 40. Scale bar, 50 μm. ( d ) Representative flow cytometry plots for analyses of TYR + cells after cells were reprogrammed by SM GFP P3 by day 100. 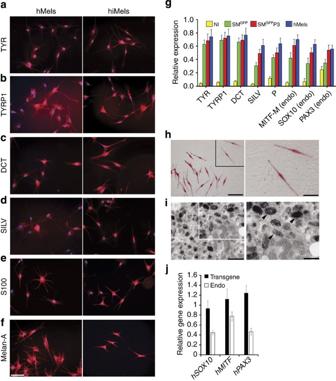Figure 4: Characterization of directly reprogrammed human iMels from fetal dermal fibroblasts. (a–f) Immunostaining analysis of human iMels (hiMels) derived from fetal hFs and normal human skin melanocytes (hMels) using antibodies specific for TYR(a), TYRP1 (b), DCT (c), SILV (d), S100 (e) and Melan-A (f). The secondary antibody was labelled with Alexa Fluro 594. DAPI was used to stain the nuclear DNA. Scale bar, 20 μm. (g) qRT–PCR analysis of melanocytic specific markers in fetal hFs infected with vector virus only (NI), SMGFPand SMGFPP3 and hMels. Melanocytic markers includedTYR,TYRP1,DCTandSILV, and endogenousSOX10,MITFandPAX3. Data shown here are mean±s.d. of the expression from three independent experiments. (h) Fontana–Masson staining showed melanin pigments in hiMels. Scale bars, 25 μm in left panel and 10 μm in right panel. Arrow heads point to the melanin pigment. (i) Electron microscopy images of hiMels with many mature melanosomes in the cytoplasm. II, stage II melanosome; III, stage III melanosome; IV, stage IV melanosome. Scale bars, 800 nm in left panel and 400 nm in right panel. Arrow heads point to melanosomes. (j) qRT–PCR analysis of transgenic and endogenous (Endo) expressions of humanPAX3(hPAX3), humanSOX10(hSXO10) and humanMITF(hMITF) in hiMels. Data shown are mean±s.d. of the expression from three independent experiments. Full size image Figure 4: Characterization of directly reprogrammed human iMels from fetal dermal fibroblasts. ( a – f ) Immunostaining analysis of human iMels (hiMels) derived from fetal hFs and normal human skin melanocytes (hMels) using antibodies specific for TYR( a ), TYRP1 ( b ), DCT ( c ), SILV ( d ), S100 ( e ) and Melan-A ( f ). The secondary antibody was labelled with Alexa Fluro 594. DAPI was used to stain the nuclear DNA. Scale bar, 20 μm. ( g ) qRT–PCR analysis of melanocytic specific markers in fetal hFs infected with vector virus only (NI), SM GFP and SM GFP P3 and hMels. Melanocytic markers included TYR , TYRP1 , DCT and SILV , and endogenous SOX10 , MITF and PAX3 . Data shown here are mean±s.d. of the expression from three independent experiments. ( h ) Fontana–Masson staining showed melanin pigments in hiMels. Scale bars, 25 μm in left panel and 10 μm in right panel. Arrow heads point to the melanin pigment. ( i ) Electron microscopy images of hiMels with many mature melanosomes in the cytoplasm. II, stage II melanosome; III, stage III melanosome; IV, stage IV melanosome. Scale bars, 800 nm in left panel and 400 nm in right panel. Arrow heads point to melanosomes. ( j ) qRT–PCR analysis of transgenic and endogenous (Endo) expressions of human PAX3 ( hPAX3 ), human SOX10 ( hSXO10 ) and human MITF ( hMITF ) in hiMels. Data shown are mean±s.d. of the expression from three independent experiments. 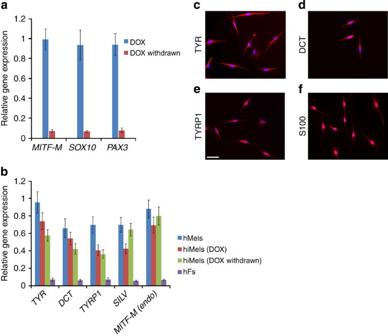Figure 5: Generation of hiMels using inducible system. HumanMITF-M,SOX10andPAX3were subcloned into doxycycline-inducible viral vectors. Fetal hFs were infected with viruses carrying these three transgenes. (a) qRT–PCR analysis of the transgenic expression ofSOX10,MITFandPAX3in the presence or absence of DOX. (b) qRT–PCR analysis of melanocytic markers in hiMels, which were stopped treating by DOX (DOX withdrawn), hiMels with DOX persistent induction (DOX), hMels and fetal hFs. hMels and fetal hFs here were used as positive and negative controls, respectively. Data shown are mean±s.d. of the expression from three independent experiments. (c–f) Immunostaining analysis of melanocytic markers including TYR (c), DCT (d), TYRP1 (e) and S100 (f) in hiMels that showed no transgenicSOX10,MITFandPAX3expression without treating by DOX. Scale bar, 30 μm. Full size image Figure 5: Generation of hiMels using inducible system. Human MITF-M , SOX10 and PAX3 were subcloned into doxycycline-inducible viral vectors. Fetal hFs were infected with viruses carrying these three transgenes. ( a ) qRT–PCR analysis of the transgenic expression of SOX10 , MITF and PAX3 in the presence or absence of DOX. ( b ) qRT–PCR analysis of melanocytic markers in hiMels, which were stopped treating by DOX (DOX withdrawn), hiMels with DOX persistent induction (DOX), hMels and fetal hFs. hMels and fetal hFs here were used as positive and negative controls, respectively. Data shown are mean±s.d. of the expression from three independent experiments. ( c – f ) Immunostaining analysis of melanocytic markers including TYR ( c ), DCT ( d ), TYRP1 ( e ) and S100 ( f ) in hiMels that showed no transgenic SOX10 , MITF and PAX3 expression without treating by DOX. Scale bar, 30 μm. Full size image Next we performed sphere formation assays to test the presence of adult stem cells in primary fetal fibroblasts in the current melanocyte culture condition. We found that passage 0 (P0) primary fetal dermal fibroblasts can form some spheres; however, passage 2 (p2) fetal fibroblasts formed few spheres and these fibroblasts were used in the melanocyte induction experiments ( Supplementary Fig. 8 ). To exclude the possibility that contaminating dermal adult stem cells or melanocyte stem cells in the fetal fibroblast cultures contributed to melanocyte induction, we cultured P2 fetal fibroblasts in the induction medium for 40 days. After this incubation period, we did not detect any cells that expressed TYR, TYRP1, DCT or Melan-A ( Supplementary Fig. 9a ). Similarly, flow cytometric analysis showed few TYR + or TYRP1 + cell populations in the culture ( Supplementary Fig. 9b ). To further clarify the purity and identity of the starting fibroblast population, we used a fibroblast marker, PDGFRA [23] , to purify fibroblasts and a melanocyte marker, c-Kit, to gate out melanocytes using the MACS MicroBead technology ( Fig. 6a ). First, we found that the PDGFRA + /c-KIT − fibroblasts formed few spheres ( Fig. 6b ). The P2 PDGFRA + /c-KIT − -purified fibroblasts were then reprogrammed by the human SM GFP P3 factors’ group. Expression of melanocytic markers was confirmed by qRT–PCR and immunostaining ( Fig. 6c,d ). These results further support that iMels are reprogrammed from dermal fibroblasts. 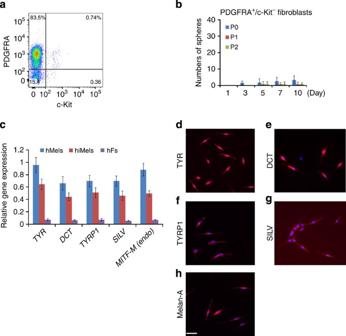Figure 6: Characterization of hiMels induced from purified human fetal fibroblasts. Human fetal PDGFRA+/c-Kit−fibroblasts were reprogrammed using SMGFPP3. (a) Flow cytometric analysis of the percentage of PDGFRA+and c-Kit+cells in primary human fetal fibroblasts. Representative data are from three independent experiments. (b) Sphere formation capacity of PDGFRA+/c-Kit−fibroblasts from primary fetal fibroblasts. P0 fibroblasts were MACS microbeads purified using an antibody against PDGFRA (positive selection) and c-Kit (negative selection). PDGFRA+/c-Kit−fibroblasts were experimented in the sphere formation assays. P0 indicates passage 0, P1 indicates passage 1 and P2 indicates passage 2. Representative data are from three independent experiments. (c) qRT–PCR analysis of melanocytic markers in hMels, hiMels derived from human fetal PDGFRA+/c-Kit−fibroblasts (hiMels) and human fetal PDGFRA+/c-Kit−fibroblasts (hFs). Data shown here are mean±s.d. of gene expression from three independent experiments. (d–h) Immunostaining analysis of melanocytic markers in hiMels including TYR (d), DCT (e), TYRP1 (f), SILV (g) and Melan-A (h). Scale bar, 30 μm. Figure 6: Characterization of hiMels induced from purified human fetal fibroblasts. Human fetal PDGFRA + /c-Kit − fibroblasts were reprogrammed using SM GFP P3. ( a ) Flow cytometric analysis of the percentage of PDGFRA + and c-Kit + cells in primary human fetal fibroblasts. Representative data are from three independent experiments. ( b ) Sphere formation capacity of PDGFRA + /c-Kit − fibroblasts from primary fetal fibroblasts. P0 fibroblasts were MACS microbeads purified using an antibody against PDGFRA (positive selection) and c-Kit (negative selection). PDGFRA + /c-Kit − fibroblasts were experimented in the sphere formation assays. P0 indicates passage 0, P1 indicates passage 1 and P2 indicates passage 2. Representative data are from three independent experiments. ( c ) qRT–PCR analysis of melanocytic markers in hMels, hiMels derived from human fetal PDGFRA + /c-Kit − fibroblasts (hiMels) and human fetal PDGFRA + /c-Kit − fibroblasts (hFs). Data shown here are mean±s.d. of gene expression from three independent experiments. ( d – h ) Immunostaining analysis of melanocytic markers in hiMels including TYR ( d ), DCT ( e ), TYRP1 ( f ), SILV ( g ) and Melan-A ( h ). Scale bar, 30 μm. Full size image Molecular characterization of hiMels Global expression analysis showed that hiMels clustered with human adult melanocytes rather than with the parental fibroblasts, as illustrated by unsupervised hierarchical clustering ( Fig. 7a ). Of note, many representative genes encoding rate-limiting enzymes for pigmented melanin production (such as TYR , TYRP1 and DCT ) were upregulated in hiMels ( Fig. 7b ). In addition, Melan-A was highly expressed in hiMels ( Fig. 7b ). Moreover, we analysed the MSigDB gene set collection for its enrichment in both hiMels and hMels. As shown in Fig. 7c , hiMels derived from human fibroblasts gained the characteristic of melanocytes (KEGG_LYSOSOME gene set and DACOSTA_UV_RESPONSE _VIA_ ERCC3 pathways) and lost the expression of fibroblast-specific gene network (MILI_PSEUDOPODIA_HAPTOTAXIS_DN and MILI_PSEUDOPODIA_ CHEMOTAXIS _DN pathways [24] ). 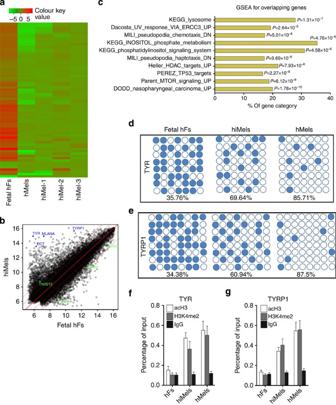Figure 7: Molecular characterization of induced human melanocytes. (a) Heatmap of genes differentially expressed in RNA microarray analysis performed on human fetal fibroblasts (fetal hFs), iMels derived from human fetal fibroblast (hiMels) and normal skin melanocytea (hMels). (b) Scatter plots show that melanocytic markers are expressed in hiMels, but not in fetal hFs. (c) Gene set enrichment analysis for the overlapping genes between hMels and hiMels. Many gene sets including KEGG_LYSOSOME, DACOSTA_UV_RESPONSE_VIA_ERCC3, PARENT_MTOR_SIGNALING_UP, MILI_PSEUDOPODIA_HAPTOTAXIS_DN and MILI_PSEUDOPODIA_CHEMOTAXIS_DN were enriched in hiMels and hMels. (d,e) DNA methylation analysis of the promoters ofTYR(d) andTYRP1(e) in fetal hFs, hiMels and hMels. Open circles indicate unmethylated CpG dinucleotides, while closed circles indicate methylated CpGs. (f,g) Histone modification analysis of promoters ofTYRandTYRP1in fetal hFs, hiMels and hMels. Chromatin immunoprecipitation was performed using antibodies against dimethylated histone H3K4 (H3K4me2) and H3 acetylation (acH3).TYRandTYRP1promoters showed enrichment for the active states (H3K4 me2 and acH3) in hiMels and hMels. In fetal hFs,TYRandTYRP1promoters appeared in the inactive state. Representative data are from three independent experiments. Figure 7: Molecular characterization of induced human melanocytes. ( a ) Heatmap of genes differentially expressed in RNA microarray analysis performed on human fetal fibroblasts (fetal hFs), iMels derived from human fetal fibroblast (hiMels) and normal skin melanocytea (hMels). ( b ) Scatter plots show that melanocytic markers are expressed in hiMels, but not in fetal hFs. ( c ) Gene set enrichment analysis for the overlapping genes between hMels and hiMels. Many gene sets including KEGG_LYSOSOME, DACOSTA_UV_RESPONSE_VIA_ERCC3, PARENT_MTOR_SIGNALING_UP, MILI_PSEUDOPODIA_HAPTOTAXIS_DN and MILI_PSEUDOPODIA_CHEMOTAXIS_DN were enriched in hiMels and hMels. ( d , e ) DNA methylation analysis of the promoters of TYR ( d ) and TYRP1 ( e ) in fetal hFs, hiMels and hMels. Open circles indicate unmethylated CpG dinucleotides, while closed circles indicate methylated CpGs. ( f , g ) Histone modification analysis of promoters of TYR and TYRP1 in fetal hFs, hiMels and hMels. Chromatin immunoprecipitation was performed using antibodies against dimethylated histone H3K4 (H3K4me2) and H3 acetylation (acH3). TYR and TYRP1 promoters showed enrichment for the active states (H3K4 me2 and acH3) in hiMels and hMels. In fetal hFs, TYR and TYRP1 promoters appeared in the inactive state. Representative data are from three independent experiments. Full size image We next analysed the DNA methylation status of TYR and TYRP1 promoters, as indicators of gene activation. As expected, TYR and TYRP1 promoters were highly demethylated in hiMels (percentage of demethylation: TYR, 69.64%; TYRP1, 60.94%) and human melanocytes (percentage of demethylation: TYR, 85.71%; TYRP1, 87.5%), whereas these same regions were highly methylated in the parental fibroblasts (percentage of demethylation: TYR, 35.67%; TYRP1, 34.38%; Fig. 7d,e ). We then performed chromatin immunoprecipitation assays to analyse histone modifications in TYR and TYRP1 promoter regions. We found that hiMels and hMels showed high levels of H3K4me2 methylation and acH3 acetylation, compared with hiMels’ parental fibroblasts ( Fig. 7f,g ). Functional characterization of hiMels in vitro and in vivo To study the biological functions of hiMels, we generated three-dimensional (3D) organotypic skin equivalents using hiMels, parental fetal fibroblasts and foreskin keratinocytes as previously described [25] . Melan-A- and S100-positive melanocytes were found to locate near the dermal–epidermal junction ( Supplementary Fig. 10a ). Fontana–Masson staining showed melanin pigment in the basal and supra-basal layer of keratinocytes, indicating that the iMels produce pigment and also transfer pigment to surrounding keratinocytes ( Supplementary Fig. 10a ). In addition, we found that melanin production in hiMels-constituted 3D skin reconstruct increased on alpha-melanocyte-stimulating hormone (α-MSH) stimulation ( Supplementary Fig. 10b ). To investigate the in vivo function of hiMels, we developed a novel assay to assess skin and hair pigmentation using a modified skin reconstitution assay [26] , [27] , [28] . In this assay, hiMels were mixed with epithelial cells and dermal fibroblasts derived from neonatal BALB/c albino mouse skin and then transplanted into the back skin of nude mice. Human normal skin melanocytes were used as positive controls. When human normal skin melanocytes or hiMels were mixed with cells prepared from BALB/c albino mouse skin, pigmented hair follicles formed ( Fig. 8a , middle and right panels). To avoid the possibility of contaminating melanocytes or melanocyte stem cells in the parental fibroblasts, we mixed parental fibroblasts with BALB/c-derived epithelial cells and dermal fibroblasts and then transplanted the cell mixture into the back skin of nude mice. Only white hair was produced under these conditions ( Fig. 8a , left panel). The grafts were harvested and histologic examination revealed epidermal-lined cysts with many hair follicles ( Fig. 8b ). We found that hiMel specifically recognized by Alu -probe labelling with fluorescein isothiocyanate were localized near the dermal–epidermal junction, inside the hair follicles and in the dermis ( Fig. 8b ). DCT + cells can be seen in the interfollicular dermis and bulb region of hair follicles ( Fig. 8c ). Meanwhile, TYRP1 + cells were observed in hair follicles and the epidermis ( Fig. 8d ). Similarly, S100 + cells were seen near the dermal–epidermal junction in the epidermis and in the hair follicles ( Fig. 8e ). We then performed Fontana–Masson staining to study the distribution of melanin pigment in the regenerated epidermis and hair follicles. Melanin pigment was detected in the epidermis, hair follicle epithelium and hair shafts ( Fig. 8f ), indicating that the hiMels were able to transfer pigment to the surrounding keratinocytes in vivo ( Fig. 8f ). The pigmentation patterns formed in the skin reconstitution assays using hiMels were identical to those of normal skin melanocytes. We did not find any melanin pigment in the skin reconstitution assays using parental fibroblasts ( Fig. 8f ). These data indicate that hiMels are functionally identical to normal skin melanocytes. 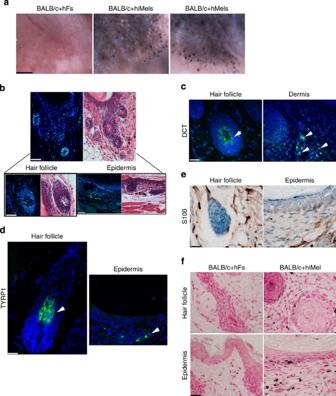Figure 8: Functional analysis of induced human melanocytesin vivo. (a) Skin reconstitution assays showed pigmented hair follicles using hiMels. hiMels, hMels or fetal hFs combined with neonatal mouse dermal fibroblasts and epithelial cells derived from BALB/c (albino) mouse skin. Cells were injected into the back skin of an immunodeficient mouse. After 3 weeks, grafts were photographed from the underside of the skin. Pigmented hair follicles were observed in hiMels or hMels groups in the skin reconstitution assays, whereas pigmented hair follicles were not observed in the group containing fetal hFs. Scale bar, 5 mm.n=5. (b) Human-specific Alu staining (green nuclei) confirmed human origin of iMels (left, upper panel) and H&E staining of consecutive section showed a cyst with hair follicle formation (right, upper panel). Scale bar, 200 μm. Human cells located in the bulb region of a hair follicle (left, lower panel) and basal layer of epidermis (right, lower panel). Scale bar, 50 μm. (c,d) Immunostaining of the xenografts from the patch assays using antibodies against human DCT (c) and TYRP1 (d). DCT+cells were present in the interfollicular dermis and bulb region of hair follicles. TYRP1+cells were observed in both hair follicles and the epidermis. Scale bar, 20 μm. (e) Immunohistochemical staining of the xenografts using the antibody against human S100. S100+-positive cells were located in epidermis, hair follicle and the dermis. Scale bar, 20 μm. (f) Fontana–Masson staining of the xenografts showed no pigments in xenografts formed by fetal hFs and mouse cells (left), whereas abundant melanin pigment was evident in the epidermis and follicular epithelium when hiMels were included in the assays (right). Scale bar, 20 μm. Figure 8: Functional analysis of induced human melanocytes in vivo . ( a ) Skin reconstitution assays showed pigmented hair follicles using hiMels. hiMels, hMels or fetal hFs combined with neonatal mouse dermal fibroblasts and epithelial cells derived from BALB/c (albino) mouse skin. Cells were injected into the back skin of an immunodeficient mouse. After 3 weeks, grafts were photographed from the underside of the skin. Pigmented hair follicles were observed in hiMels or hMels groups in the skin reconstitution assays, whereas pigmented hair follicles were not observed in the group containing fetal hFs. Scale bar, 5 mm. n =5. ( b ) Human-specific Alu staining (green nuclei) confirmed human origin of iMels (left, upper panel) and H&E staining of consecutive section showed a cyst with hair follicle formation (right, upper panel). Scale bar, 200 μm. Human cells located in the bulb region of a hair follicle (left, lower panel) and basal layer of epidermis (right, lower panel). Scale bar, 50 μm. ( c , d ) Immunostaining of the xenografts from the patch assays using antibodies against human DCT ( c ) and TYRP1 ( d ). DCT + cells were present in the interfollicular dermis and bulb region of hair follicles. TYRP1 + cells were observed in both hair follicles and the epidermis. Scale bar, 20 μm. ( e ) Immunohistochemical staining of the xenografts using the antibody against human S100. S100 + -positive cells were located in epidermis, hair follicle and the dermis. Scale bar, 20 μm. ( f ) Fontana–Masson staining of the xenografts showed no pigments in xenografts formed by fetal hFs and mouse cells (left), whereas abundant melanin pigment was evident in the epidermis and follicular epithelium when hiMels were included in the assays (right). Scale bar, 20 μm. Full size image To test whether MITF alone is sufficient to generate functional melanocytes in vivo , we cultured MITF-infected fibroblasts for 50 days in the melanocyte-inducing medium. We then transplanted MITF-infected fibroblasts with BALB/c-derived epithelial cells and dermal fibroblasts’ mixture to mouse back skin. We did not find any pigment in the hair follicles and epidermis in the skin reconstruct ( Supplementary Figs 11a,b ), indicating that MITF alone is insufficient to convert fibroblast to melanocyte. Direct reprogramming of human adult dermal fibroblasts into iMels We then used the same procedure to human adult fibroblasts (adult hFs) and infected them with the SM GFP P3 virus combination. The SM GFP P3-infected cells were cultured for 15 days, and GFP + cells were then sorted and cultured in melanocyte-inducing medium for 40 days. qRT–PCR analysis of the GFP + cells showed the activated melanocytic network for melanin production and transfer ( Supplementary Fig. 12a ). We also detected that key melanocytic markers including TYR, DCT, S100 and Melan-A were expressed in cells with typical melanocyte morphology ( Supplementary Fig. 12b ). Notably, only 6% of the adult hFs expressed melanocytic markers, indicating that the adult fibroblast-reprogramming efficiency was much lower than that for fetal fibroblasts ( Supplementary Fig. 12c ). We performed flow cytometric analysis to measure the percentage of the TYR + and TYRP1 + cells in the adult reprogrammed cells and found only 3.27 and 2.16%, respectively ( Supplementary Fig. 12d ). Our results demonstrate that SOX10, MITF and PAX3 are sufficient to reprogram mouse and human fibroblasts into functional melanocytes. iMels generated using our method acquire all the biochemical and functional characteristics of normal melanocytes. Substantial progress has been achieved with the discovery of transdifferentiation of somatic cells to other lineage-specific cell types [4] , [5] , [7] , [8] , [9] , [10] , [11] , [29] , suggesting that somatic cell fates can be interconverted without transiting through distinct hierarchies. We previously showed that a multipotent cell population in the foreskin dermis can be differentiated into melanocytes [30] . However, this approach is limited by the small percentage (0.085%) of dermal stem cells present in foreskin and the relatively low differentiation efficiency of these cells to melanocytes. In addition, the foreskin dermal stem cell population gradually disappears with serial passage. To exclude the possibility that these dermal stem cells contributed to melanocyte direct reprogramming, we used a fibroblast cell surface marker, PDGFRA [23] , to sort out PDGFRA + /c-Kit − fibroblasts. We showed that these purified fibroblasts can also be reprogrammed into melanocytes, supporting that iMels are directly reprogrammed from dermal fibroblasts. Nevertheless, despite our extensive efforts to characterize the starting dermal fibroblasts, we cannot completely exclude the possibility that some of the iMels might be derived from multipotent cells in the dermis. In translational medicine, generation of functional melanocytes by direct reprogramming establishes a means for obtaining a scalable source of autologous melanocytes, which then could be used for developing cell-based treatments for pigmentary disorders such as vitiligo and hypopigmentation associated with congenital disorders. Reprogramming fibroblasts into melanocytes specifically from patients with melanoma also serves as a powerful strategy for studying the aetiology of melanoma. Cell culture TTFs were isolated from the Tyrosinase-CreER / Gt (ROSA)26Sor tm4(ACTB-tdTomato,-EGFP)Luo /J transgenic and C57BL/6 mice. Tails were peeled, minced into 1 cm pieces, placed on culture dishes and incubated in MEF media (Dulbecco’s modified Eagle medium (DMEM; Invitrogen) containing 10% fetal bovine serum (FBS; Hyclone), non-essential amino acids (Invitrogen), sodium pyruvate and penicillin/streptomycin (Invitrogen)) for 5 days. MEFs were isolated from day 14.5 mouse embryos. Cells were split no more than three times in all experiments. Human fetal fibroblasts were isolated from 20-week-old fetal skin (Advanced Bioscience Resources; Alameda, CA). Adult hFs were obtained from discarded normal skin after surgery following a protocol approved by the University of Pennsylvania Institutional Review Board. Human skin samples were mechanically dissociated, plated on gelatin-coated dishes and cultured in MEF media. XB2, an immortal line of mouse keratinocytes, was cultured in MEF media. HEK 293T cells and human fibroblasts were cultured in DMEM supplemented with 10% FBS, 2 mM L -glutamine, 100 U ml −1 penicillin and 100 μg ml −1 of streptomycin (all from Invitrogen). Viral infection For mouse cell infection, viruses were packaged by transfecting retroviruses and pECO into 293T cells. For human cell infection, pantropic viruses were packaged by transfecting the retrovirus vectors, pUMVC and pCMV-VSVG into 293T cells. To improve the pantropic retrovirus infection efficiency, we concentrated the virus using the Retro-X Concentrator (Clontech) according to manufacturer’s instruction. After 48 h, growth medium was replaced with mouse melanocyte-inducing medium containing RPMI 1640 (Invitrogen), 10% FBS, 10 ng ml −1 basic fibroblast growth factor (bFGF) (Invitrogen), 100 ng ml −1 SCF (R&D), 100 nM ET-3 (American Peptide Company), 20 pM cholera toxin (CT) (Sigma-Aldrich) and 200 nM 12-O-tetradecanoyl-phorbol 13-acetate (TPA; Sigma-Aldrich). Human melanocyte-inducing medium contained medium 254, 10 ng ml −1 bFGF, 100 ng ml −1 stem cell factor (SCF) and 100 nM ET-3. For G418 selection, 60 μg ml −1 G418 was added to melanocyte-induction media. Flow cytometry and cell sorting Cells (2.5 × 10 6 cells ml −1 ) were stained with antibodies against TYR (Abcam), TYRP1 (Sigma), c-Kit (eBioscience) and PDGFRA (BioLegend). To detect intracellular proteins, staining was carried out on cells fixed with 4% paraformaldehyde (Electron Microscopy Sciences) in PBS. Staining was performed in PBS with 2% FBS. Stained cells and GFP + cells were analysed using an LSRII flow cytometer (BD). For FACS sorting, cells were sorted at a concentration of 10 6 cells ml −1 in PBS/2% FBS using a FACSAriaTMII (BD) cell sorter (Upenn Flow Cytometry Facility). PDGFRA + /c-Kit − fibroblasts were sorted from P1 fetal hFs and cultured as P0. For magnetic bead sorting, the Miltenyi MACS bead sorting system was used according to the manufacturer’s guidelines. Data were analysed using FlowJo software (Treestar). The working solutions of antibodies are shown in Supplementary Table 3 . Immunofluorescence and immunochemistry Monolayer cells were fixed with 4% paraformaldehyde and stained with primary antibodies specific for TYR, TYRP1, DCT (polyclonal; a gift from Dr V.J. Hearing, Bethesda, MD), Melan-A, SILV and S100 (polyclonal; Dako). After washing, cells were incubated with the appropriate Alexa Fluor 594-labelled secondary antibodies (Invitrogen). Paraffin-embedded slides were deparaffinized, followed by antigen retrieval and staining as described above. Immunofluorescence for DCT was performed as described above. Immunohistochemical staining for S100, melan-A and Fontana–Masson was performed on paraffin-embedded slides using standard immunoperoxidase techniques. The working solutions of antibodies are shown in Supplementary Table 3 . Quantitative RT–PCR RNA was extracted from single cultures using RNA mini kits (Qiagen) according to manufacturer’s instructions. We performed reverse transcription reactions using SuperScript III First-Strand Synthesis Kit (Invitrogen). qPCR was performed using SYBR Green Supermix (Bio-Rad) and reactions were analysed using the Bio-Rad qPCR detection system. The primers used are listed in Supplementary Table 2 . Global gene profiling and array analysis Microarray raw data generated from Illumina Chips were normalized, background corrected and summarized using the R package ‘lumi’ [31] . To reduce false positives, unexpressed probes were removed from analysis and 21,758 probes were examined in all experiments described herein. The R package ‘limma’ [32] , [33] was used to evaluate differential gene expression analysis, followed by multiple test correction by the Benjamini and Hochberg procedure 37 (ref. 34 ). The genes with the adjusted P values <0.05 and fold changes >4 were subjected to the two-way clustering analysis to generate the heatmaps. Gene set enrichment analysis analysis was performed as described previously [35] . Briefly, the top-bound genes in the iMel and parental Fibroblast data sets were selected, and the overlapping genes were subjected to analysis by using the MSigDB gene set collection. Bisulfite genomic sequencing Bisulfite treatment was performed using the CpGenome modification Kit (Millipore) according to the manufacturer’s recommendations. The PCR primers used are listed in the Supplementary Table 2 . Amplified products were cloned into pCR2.1-TOPO (Invitrogen). Ten randomly selected clones were sequenced with the M13 forward and M13 reverse primers for each gene. Sequencing was performed at the University of Pennsylvania sequencing facility. CpG methylation of the sequence was analysed by BiQ Analyzer software. Chromatin immunoprecipitation A total of 10 7 hFFs, hiMels or human melanocytes were fixed with 1% formaldehyde at room temperature for 10 min and then lysed in 1 ml lysis buffer (50 mM Tris-HCl, pH 8.0, 10 mM EDTA, 1% SDS and protease inhibitors) on ice for 20 min. The lysate was split into three tubes and sonicated. After 10 min centrifugation, the supernatant was pre-cleared by incubating at 4 °C for 4 h with agarose beads pre-blocked with BSA (1 mg BSA for 10 ml beads) in immunoprecipitation buffer (50 mM Tris-HCl, pH 8.0, 150 mM NaCl, 2 mM EDTA, 1% NP-40, 0.5% sodium deoxycholate, 0.1% SDS and protease inhibitors). A total of 100 μl of pre-cleared chromatin diluted in 1 ml IP buffer in the presence of 20 μg antibody was used for each immunoprecipitation reaction according to the manufacturer’s protocol. The antibodies used for this study were: anti-acH3 (Millipore), anti-dimethyl K4 of H3 (H3K4me2, Millipore) and normal rabbit IgG (Sigma). The precipitate was purified and analysed by qPCR. PCR primers are listed in Supplementary Table 2 . Sphere formation assay Sphere formation assay was performed as described previously [36] . Briefly, dissociated cells were plated in serum-free media in low-cell-density cultures with exogenous growth factors used at final concentrations of 10 ng ml −1 bFGF and 100 ng ml −1 SCF. Sphere colonies were generated and counted under the microscope. Human 3D skin reconstructs Human 3D skin reconstructs were generated as described previously [25] . Briefly, inserts of tissue culture trays (Organogenesis, Canton, MA) were coated with 1 ml bovine collagen I (Organogenesis) and layered with 3 ml collagen I containing 7.5 × 10 4 fibroblasts. After 4–7 days at 37 °C, hiMels were mixed with keratinocytes and seeded on top of the dermal reconstructs at a ratio of 1:5 (hiMels to keratinocytes). After 4 days, human keratinocytes were added and the cells were cultured in skin reconstruct media: keratinocyte serum-free medium (Invitrogen) with 60 μg ml −1 bovine pituitary extract, 2% dialysed FBS (Invitrogen), 4.5 ng ml −1 bFGF (Invitrogen), 100 nM ET-3 (sigma) and 10 ng ml −1 SCF (R&D system). Cultures were submerged in media containing 1 ng ml −1 epidermal growth factor (EGF; Invitrogen) for 2 days, 0.2 ng ml −1 EGF for another 2 days, then maintained at the air–liquid interface and incubated in high-calcium (2.4 mM) media. Two weeks later, skin reconstructs were harvested, fixed in 10% neutral buffered formalin for 3 h and processed by routine histological methods. For α-MSH treatment assay, 50 nM α-MSH was added to induce the melanin production in the cultured reconstructed skin. Pigmented skin reconstitution assays with melanocytes The protocol has been approved by the University of Pennsylvania Institutional Animal Care and Use Committee. Skin reconstitution assays were performed as described previously [27] , [28] . Briefly, truncal skin from 1-day postnatal BALB/c mice, a mouse strain with non-pigmented white hair coat, was removed and rinsed in free PBS. The skin was laid flat in PBS containing dispase (2.5 mg ml −1 , Invitrogen) at 4 °C overnight. Inductive dermal cells and epidermal cells were isolated as previously described [37] , [38] , [39] . In brief, epidermis and dermis were separated first. Epidermal and dermal cells were then isolated for skin reconstitution. Trichogenic cells were assayed in male nude (nu/nu) mice (Charles River) at 7–9 weeks. For each intracutaneous injection, 1 × 10 6 BALB/c neonatal dermal cells and 10,000 epidermal aggregates were used. To test the ability of hiMels to participate in the formation of hair follicles and produce pigmented shafts in the reconstitution assay, 0.5 × 10 6 hiMels were added to the neonatal BALB/c dermal and epidermal cell mixture for each injection. As positive controls, 0.5 × 10 6 cultured human melanocytes were added in separate injections with the mouse cells. The cell mixtures were resuspended in 50–70 μl of DMEM-F12 medium (Invitrogen) and injected (25-gauge needle) into the hypodermis of the mouse skin, forming a bleb. The injection site was marked by a black tattoo puncture (242 Permanent Black Pigment, Aims, Hornell, New York). The skin reconstruct was harvested at 2 weeks after injection and the newly formed hair follicles were examined under a dissection microscope. Two independent experiments with different batches of hiMels were performed, with two duplicate sets each time. In situ hybridization Briefly, paraffin slides were dehydrated, antigen retrieved and hybridized with Alu DNA probe (BioGenex PR-1001-01, ready to use): heat slide at 85 °C for 10 min and then incubate at 37 °C overnight. The slides were then incubated with antibody specific for fluorescein, biotin labelled (BioGenex AS2505-16, ready to use) and finally incubated with secondary antibody labelled with Streptavidin-Alexa Fluo 488. DAPI (4',6-diamidino-2-phenylindole) was used to label nuclear DNA. Statistical analysis Student’s t -test or analysis of variance was used to analyse gene expression and flow cytometric data. qPCR data were analysed after being normalized for β-actin loading control. Error bars indicate s.d. Statistical significance was determined if two-sided P <0.05. How to cite this article: Yang, R. et al. Direct conversion of mouse and human fibroblasts to functional melanocytes by defined factors. Nat. Commun. 5:5807 doi: 10.1038/ncomms6807 (2014). Accession codes: Microarray data has been deposited in Gene Expression Omnibus under accession number GSE51028 .